Early selection ofbZIP73facilitated adaptation ofjaponicarice to cold climates Cold stress is a major factor limiting production and geographic distribution of rice ( Oryza sativa ). Although the growth range of japonica subspecies has expanded northward compared to modern wild rice ( O. rufipogon ), the molecular basis of the adaptation remains unclear. Here we report bZIP73 , a bZIP transcription factor-coding gene with only one functional polymorphism (+511 G>A) between the two subspecies japonica and indica , may have facilitated japonica adaptation to cold climates. We show the japonica version of bZIP73 (bZIP73 Jap ) interacts with bZIP71 and modulates ABA levels and ROS homeostasis. Evolutionary and population genetic analyses suggest bZIP73 has undergone balancing selection; the bZIP73 Jap allele has firstly selected from standing variations in wild rice and likely facilitated cold climate adaptation during initial japonica domestication, while the indica allele bZIP73 Ind was subsequently selected for reasons that remain unclear. Our findings reveal early selection of bZIP73 Jap may have facilitated climate adaptation of primitive rice germplasms. Rice ( Oryza sativa ) is one of the most important cereal crops feeding more than half of the world’s population [1] , [2] . As a tropical plant, rice is more sensitive to cold stress than other cereal crops such as wheat ( Triticum aestivum ) and barley ( Hordeum vulgare ) [3] , [4] . Therefore, in high-latitude and high-altitude regions, cold stress is a major limiting factor for rice growth and production [3] , [5] , [6] . Asian rice consists of two geographically and genetically diverged subspecies, indica and japonica , which are distinct in their ability to tolerate cold stress [7] , [8] , [9] . In general, japonica cultivars are more cold tolerant than indica and predominate temperate zones (e.g., northern China, Korea, and Japan), whereas indica cultivars grow in tropical and subtropical regions (e.g., southern China and South Asia) [10] . Despite the divergence of rice cultivars, the domestication history of cultivated rice is uncertain due to contrasting evidences. Garris et al. [11] revealed the deep genetic structure and diversity of different rice ecotypes [11] , and, based on phylogenetic studies, Londo et al. [12] and Civáň et al. [13] proposed multiple independent domestication events for cultivated rice [12] , [13] . In contrast, Huang et al. [14] and Choi et al. [15] proposed that rice was initially domesticated as japonica , while subsequent backcrosses to different groups of common wild rice ( O. rufipogon ) generated indica , aus , and other subpopulations [14] , [15] . However, two recent studies using large-scale rice populations found limited introgression signals around key domestication genes [16] , [17] . Although the common wild rice is considered the direct ancestor of modern cultivated rice, the species itself has diverged into several groups that may represent different origins of modern cultivated rice [12] , [14] , [18] , [19] . Moreover, wild rice populations did not expand to eastern and northern China until the Last Glacial Maximum ~16,000 years ago when warm and wet conditions emerged [20] . During the expansion to cold climates, positive selections on standing variations of functional genes probably facilitated rice adaptation to cold stress [21] . For example, artificial selection of a single-nucleotide polymorphism (SNP) in COLD1 , a gene regulating G-protein signaling, enhanced cold tolerance in japonica rice [21] ; and the wild rice-derived haplotype of CTB4a was retained by artificial selection during temperate japonica domestication in cold habitats [22] . Cold tolerance is a complex trait [3] . Several genes associated with cold stress have been identified so far, which can be divided into two groups. The first group consists of functional components that directly protect plant cells from cold stress, i.e., enzymes in metabolic pathways [23] . The second group consists of genes that regulate gene expression during stress responses, i.e., signaling components and transcription factors (TFs) [23] . Together with their target genes, TFs can constitute regulons that participate in signal transduction for activating or repressing genes involved in cold stress responses. Thus, TFs are excellent candidates for modification of complex traits in crops [24] . The basic leucine zipper (bZIP) family is one of the most diverse TF families in vascular plants and has 91 members in rice [25] , [26] , some of which are involved in cold stress responses [25] , [27] , [28] , [29] , [30] . For example, OsbZIP52/RISBZ5 functions as a negative regulator of cold stress tolerance [31] ; OsbZIP38/LIP19 interacts with OsbZIP87/OBF1 and plays important roles in cold signaling pathways [32] ; and a number of bZIP genes are up- or down-regulated under cold stress conditions [25] , [33] . However, a potential contribution of bZIP TFs to the northward expansion of japonica has not yet been investigated. To fill this gap, we combined association studies, population genetics, and stress-response profiling for the identification of candidate bZIP genes. Our results show that bZIP73 contributes to low-temperature seedling survivability (LTSS) and may have been a target of selection during the domestication of japonica rice. Molecular and transgenic studies revealed that the japonica version of bZIP73 (bZIP73 Jap ) interacts with bZIP71 and functions by modulating abscisic acid (ABA) level and reactive oxygen species (ROS) homeostasis, which could significantly enhance rice tolerance to cold. Evolutionary and population genetic analyses suggest that the two alleles of bZIP73 have undergone several rounds of artificial selection in both common wild rice and cultivated rice, indicating that balancing selection may have occurred on this gene. Selection of bZIP73 Jap in the direct ancestor of japonica suggests that the gene may have contributed to cold climate adaptation during the early stages of japonica domestication. bZIP73 is an excellent cold tolerance candidate gene in rice To systematically study natural variations of bZIP genes, we combined two published Oryza resequencing populations, the USDA (United States Department of Agriculture) rice mini-core population [34] and a large collection of common wild rice [14] . The combined population has a total of 641 cultivars or accessions collected from over 15 geographic regions (Supplementary Fig. 1 ) [35] , which includes 66 indica , 57 japonica , 81 other cultivars ( aus , aromatic , and admixture varieties), and 435 common wild rice strains. From the high-density SNP set (2.3 M) we previously generated for the combined population [34] , a total of 27,008 SNPs including 1010 non-synonymous substitutions were identified in the coding region of 91 bZIP genes. We measured the LTSS of the mini-core population for association analyses with the bZIP gene family [36] . Unlinked amino-acid (aa) variations were used as association markers. 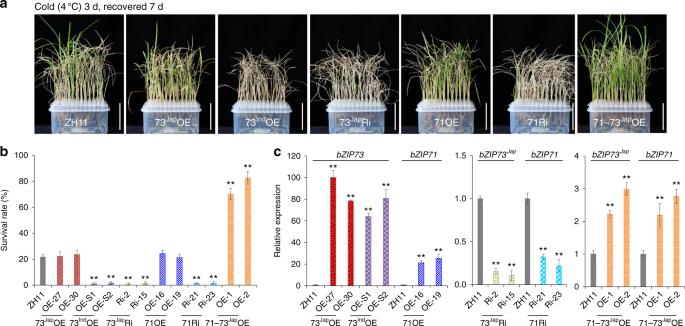Fig. 1 Assessment of cold stress tolerance ofbZIP73andbZIP71transgenic rice.aOverexpression linesbZIP73Jap(73JapOE),bZIP73Ind(73IndOE), andbZIP71(71OE), co-expression linesbZIP71-bZIP73Jap(71–73JapOE), and RNAi linesbZIP73Jap(73JapRi) andbZIP71(71Ri) were cold treated at 4 °C for 3 days and are shown after recovery at 28 °C for 7 days. ZH11, wild-type Zhonghua 11.bSurvival rates of ZH11 and transgenic lines recovered after cold treatment. Scale bars, 5 cm.cRelative expression levels ofbZIP73andbZIP71in ZH11 and transgenic lines measured by real-time PCR under normal condition. Target genes for measurement are indicated on top of the plot, and expression levels in ZH11 (wild-type plants) was used as reference (1×) to show expression fold change (y-axes) in transgenic lines as indicated onx-axes. Due to the different scale of relative expression levels, data were separated into three subplots. All data were collected using two independent homozygous lines indicated onx-axes with three biological replicates (n= 288 each). Error bar, standard deviation; **p< 0.01, two-tailedt-test in comparison to ZH11 After correcting for population structure and adjusting the false discovery rate (FDR) for multiple testing [37] , the following 8 out of 91 bZIP genes were significantly correlated with the LTSS phenotype ( p < 0.05, FDR_BH) (Supplementary Table 1 ): OsbZIP08 , OsbZIP35 , OsbZIP38 , OsbZIP46 , OsbZIP63 , OsbZIP72 , OsbZIP73 , and OsbZIP76 . The northward expansion of japonica was probably achieved by local adaptation to cold stress. We thus scanned for genomic footprints of local adaptation using a linkage disequilibrium (LD)-based ω statistics [38] . 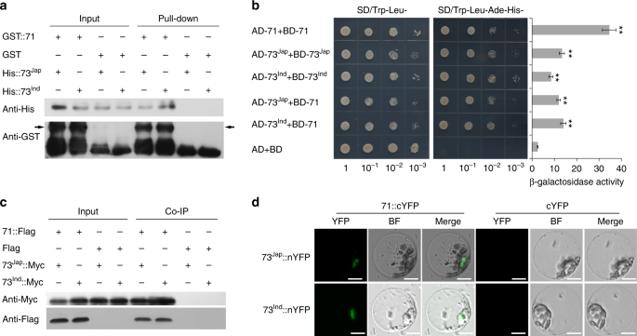Fig. 2 In vivo and in vitro interaction assays between bZIP71 and bZIP73.aIn vitro pull-down assay. Left panel (Input), 10% of input before precipitation; Right panel (Pull-down), affinity purification using glutathioneS-transferase (GST) or GST::71 as bait, and polyhistidine (His)::73Japor His::73Indas prey. Anti-His and anti-GST antibodies were used to detect His and GST peptides, respectively. Black arrows indicate anti-GST detection of GST::71, and + and − indicate that ingredients shown at the left were added or not added, respectively, to the experiment.bIn vivo yeast two-hybrid assay. Sequences of bZIP73Jap, bZIP73Ind, and bZIP71 were fused to both the pGADT7 activation domain (AD, prey) and the pGBKT7 binding domain (BD, bait), and then transformed into yeast. Shown are growth phenotypes of yeast transformants on selective media of SD/Trp-Leu- (left panel) and SD/Trp-Leu-His-Ade- (central panel, interaction). Physical protein–protein interactions were revealed by yeast colony sizes and quantified by β-galactosidase activity (right panel) using a liquid culture assay with three biological replicates. Error bar, standard deviation; **p< 0.01, two-tailedt-test in comparison to the negative control, AD (pGADT7)+BD (pGBKT7).cIn vivo co-immunoprecipitation (Co-IP) assay. Sequences of bZIP73Japand bZIP73Indwere fused with a Myc tag, while bZIP71 were fused with a Flag tag. Vectors of 73Jap::Myc and 73Ind::Myc were transformed into transgenic rice lines expressing 71::Flag. Left panel (Input), before precipitation; Right panel (Co-IP), Anti-Myc and anti-Flag antibodies were used to detect Myc and Flag peptides, respectively.dIn vivo bimolecular fluorescence complementation assay. bZIP73Japand bZIP73Indwere both fused with the N-terminal half of yellow fluorescent protein (nYFP), while bZIP71 was fused with the C-terminal half of YFP (cYFP). BF, bright field. Merge is overlay of YFP and bright field images showing nuclear localization. Right panel, negative control. Scale bars, 10 µm Of the eight LTSS-correlated bZIP genes, only bZIP73 showed excessive LD increments, indicating that a positive selection for bZIP73 occurred in japonica (Supplementary Table 2 ). These results strongly suggest that bZIP73 is an excellent candidate to investigate the japonica adaptation to a cold climate. The TF bZIP73 is diverged between japonica and indica bZIP73 ( LOC_Os09g29820 ) encodes a typical bZIP protein (173 aa) that contains a single SNP affecting the C terminus of the protein sequence (Supplementary Fig. 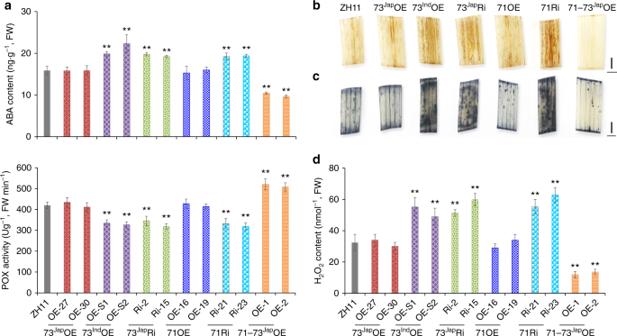Fig. 3 Metabolic responses of wild-type and transgenic rice lines under cold stress.aABA content (n= 3, 32 plants/replication) and peroxidase (POX) enzyme activity (n= 8, 10 plants/replication) of transgenic lines under cold stress.bThe 3,3’-diaminobenzidine (DAB) andcnitroblue tetrazolium (NBT) staining for the visualization of H2O2and O2−, respectively, in cold-treated rice leaves. Scale bars, 2 mm.dH2O2content (n= 8, 10 plants/replication) of transgenic lines under cold stress. OE, overexpression; Ri, RNA interference; 73Jap,bZIP73Jap; 73Ind,bZIP73Ind; 71,bZIP71; 71–73JapOE, overexpression of bothbZIP71andbZIP73Jap; FW, fresh weight. All experiments were conducted using two-week-old seedlings. Error bar, standard deviation; **p< 0.01, two-tailedt-test 2 ), which is diverged between japonica and indica (+511 bp, G>A; +171 aa, Glu>Lys; the first bp or the first aa of the coding region was defined as +1) (Supplementary Table 3 and Supplementary Data 4 ). We hereafter used the names of bZIP73 Jap and bZIP73 Ind for the japonica and indica haplotypes, respectively. Using bZIP73::GFP fusion proteins in rice protoplasts, we found that both bZIP73 versions exclusively co-localized with a nuclear marker, OsMADS3::mCherry (Supplementary Fig. 3a, b ). Truncated bZIP73 proteins (binding domain (BD)-73N2, 1–156 aa; BD-73M, 77–156 aa; BD-73 Jap/Ind C2, 77–173 aa), which contained both the basic region and leucine zipper domains, had transactivation activities in yeast (Supplementary Fig. 3c, d ). However, neither the full-length CDS (BD-73 Jap/Ind , 1–173 aa) nor smaller truncated constructs (BD-73N1, 1–99 aa, containing the basic region domain; BD-73 Jap/Ind C1, 100–173 aa, containing the leucine zipper domain) of bZIP73 had transactivation activities in yeast (Supplementary Fig. 3c, d ). These results indicate that the bZIP domain (basic region and leucine zipper) of bZIP73 is required for its transactivation activity, while the N-terminal (1–76 aa) and the C-terminal (157–173 aa) domains may be negative regulators of the transcriptional activity of bZIP73. A SNP in bZIP73 alters cold sensitivity between japonica and indica subgroups To determine whether bZIP73 was under environmental control, we analyzed its expression profile under different abiotic stresses. Transcript levels of bZIP73 increased after 1 to 6 h of cold, ABA, and H 2 O 2 treatments in roots and/or shoots of rice seedlings (Supplementary Fig. 4 ), indicating that bZIP73 may function in ABA-dependent cold signaling pathways. To further characterize the function of bZIP73 , we overexpressed bZIP73 Jap (73 Jap OE) and bZIP73 Ind (73 Ind OE) separately in the japonica cultivar Zhonghua 11 (ZH11) and silenced bZIP73 Jap (73 Jap Ri) using RNA interference (RNAi) in ZH11. Two-week-old rice seedlings of homozygous transgenic lines (T 3 generation) were exposed to cold stress (4 °C) for 3 days and subsequently returned to normal temperature (28 °C) for recovery (Supplementary Fig. 5 ). Our results showed that both 73 Ind OE and 73 Jap Ri lines were more sensitive to cold stress than the wild type (WT), because they had <2% survival rates (the percentage of recovered seedlings), which was significantly lower than the 22% survival rate of WT plants (Fig. 1a, b ) ( p < 0.01, two-tailed t- test). However, the survival rate of 73 Jap OE lines was not significantly different from that of WT plants (Fig. 1a, b ), indicating that the function of bZIP73 may require cofactors. Fig. 1 Assessment of cold stress tolerance of bZIP73 and bZIP71 transgenic rice. a Overexpression lines bZIP73 Jap (73 Jap OE), bZIP73 Ind (73 Ind OE), and bZIP71 (71OE), co-expression lines bZIP71 - bZIP73 Jap (71–73 Jap OE), and RNAi lines bZIP73 Jap (73 Jap Ri) and bZIP71 (71Ri) were cold treated at 4 °C for 3 days and are shown after recovery at 28 °C for 7 days. ZH11, wild-type Zhonghua 11. b Survival rates of ZH11 and transgenic lines recovered after cold treatment. Scale bars, 5 cm. c Relative expression levels of bZIP73 and bZIP71 in ZH11 and transgenic lines measured by real-time PCR under normal condition. Target genes for measurement are indicated on top of the plot, and expression levels in ZH11 (wild-type plants) was used as reference (1×) to show expression fold change ( y -axes) in transgenic lines as indicated on x -axes. Due to the different scale of relative expression levels, data were separated into three subplots. All data were collected using two independent homozygous lines indicated on x -axes with three biological replicates ( n = 288 each). Error bar, standard deviation; ** p < 0.01, two-tailed t -test in comparison to ZH11 Full size image bZIP73 interacts with bZIP71 and enhances cold tolerance To identify potential bZIP73 cofactors, we performed a yeast two-hybrid (Y2H) screening by using full-length CDS of bZIP73 Jap fused to pGBKT7 (BD-73 Jap ) as bait, and identified 23 potential cofactors including another bZIP protein, bZIP71 (Supplementary Data 1 ). The interaction between bZIP71 and bZIP73 Jap/Ind was further confirmed through additional Y2H assays in vitro (Fig. 2b ) and in vivo using bimolecular fluorescence complementation (BiFC) assays in rice protoplasts (Fig. 2d ). Furthermore, we performed co-immunoprecipitation (Co-IP) experiments and found that both bZIP73 Jap and bZIP73 Ind were co-immunoprecipitated with bZIP71 in vivo (Fig. 2c ). Consistent with these results, an in vitro pull-down assay also showed a direct physical interaction between bZIP73 Jap/Ind and bZIP71 (Fig. 2a ). Together, these in vitro and in vivo experiments suggest that both bZIP73 Jap and bZIP73 Ind can interact with bZIP71. Fig. 2 In vivo and in vitro interaction assays between bZIP71 and bZIP73. a In vitro pull-down assay. Left panel (Input), 10% of input before precipitation; Right panel (Pull-down), affinity purification using glutathione S -transferase (GST) or GST::71 as bait, and polyhistidine (His)::73 Jap or His::73 Ind as prey. Anti-His and anti-GST antibodies were used to detect His and GST peptides, respectively. Black arrows indicate anti-GST detection of GST::71, and + and − indicate that ingredients shown at the left were added or not added, respectively, to the experiment. b In vivo yeast two-hybrid assay. Sequences of bZIP73 Jap , bZIP73 Ind , and bZIP71 were fused to both the pGADT7 activation domain (AD, prey) and the pGBKT7 binding domain (BD, bait), and then transformed into yeast. Shown are growth phenotypes of yeast transformants on selective media of SD/Trp-Leu- (left panel) and SD/Trp-Leu-His-Ade- (central panel, interaction). Physical protein–protein interactions were revealed by yeast colony sizes and quantified by β-galactosidase activity (right panel) using a liquid culture assay with three biological replicates. Error bar, standard deviation; ** p < 0.01, two-tailed t -test in comparison to the negative control, AD (pGADT7)+BD (pGBKT7). c In vivo co-immunoprecipitation (Co-IP) assay. Sequences of bZIP73 Jap and bZIP73 Ind were fused with a Myc tag, while bZIP71 were fused with a Flag tag. Vectors of 73 Jap ::Myc and 73 Ind ::Myc were transformed into transgenic rice lines expressing 71::Flag. Left panel (Input), before precipitation; Right panel (Co-IP), Anti-Myc and anti-Flag antibodies were used to detect Myc and Flag peptides, respectively. d In vivo bimolecular fluorescence complementation assay. bZIP73 Jap and bZIP73 Ind were both fused with the N-terminal half of yellow fluorescent protein (nYFP), while bZIP71 was fused with the C-terminal half of YFP (cYFP). BF, bright field. Merge is overlay of YFP and bright field images showing nuclear localization. Right panel, negative control. Scale bars, 10 µm Full size image Similar to other known bZIP interactions [32] , [39] , we hypothesized that the bZIP73-bZIP71 interaction may facilitate activation of bZIP73 through a similar mechanism as previously reported for OsbZIP38-OsbZIP87, which confers a cold signal switch in rice [32] . To test this, we co-overexpressed bZIP73 Jap and bZIP71 in ZH11 (71–73 Jap OE) and subjected seedlings to cold stress at 4 ℃ for 3 days (Supplementary Fig. 5 ). In agreement with our hypothesis, the seedling survival rate was positively correlated with expression levels of bZIP71 and bZIP73 Jap (Fig. 1b, c ), which was greatly improved to >70%, while that of wild-type ZH11 was only 22% (Fig. 1a, b ). These results indicated that co-overexpression of bZIP71 and bZIP73 Jap significantly improves rice tolerance to cold stress ( p < 0.01, two-tailed t- test). bZIP71 enhances bZIP73 Jap activity to reduce ROS levels To further understand how bZIP73 Jap regulates cold stress tolerance, we used chromatin immunoprecipitation (ChIP) sequencing to pull-down bZIP73 Jap targets and identified 669 non-TE genes that were precipitated with bZIP73 Jap ::Flag (Supplementary Data 2 ). These genes were enriched in Gene Ontologies (GOs) of abiotic stress responses (Supplementary Fig. 6 ), including four peroxidase (POX) precursor genes ( LOC_Os01g22249 , LOC_Os03g02920 , LOC_Os03g32050 , and LOC_Os04g59210 ) that share a typical regulatory G-box motif targeted by bZIP TFs in their promoters (Supplementary Data 3 ). The interaction between bZIP73 Jap ::Flag and the promoters of these four genes were further confirmed by ChIP quantitative PCR (qPCR) (Supplementary Fig. 7b ). Transient expression assays in rice protoplasts showed that the promoter activities of these POX precursors were induced by cold treatment and enhanced by the addition of bZIP73 Jap ( p < 0.01, two-tailed t- test) (Supplementary Fig. 8 ). Excitingly, the addition of bZIP71 significantly enhanced the transcription of these POX precursors under both normal condition and cold condition ( p < 0.01, two-tailed t- test) (Supplementary Fig. 8 ). POXs are involved in defense against abiotic stresses through scavenging of ROS [40] , [41] . We found that both the expression of POX precursor genes and the POX activity were significantly up-regulated in 71–73 Jap OE lines after cold stress (4 °C, 3 h) (Fig. 3a and Supplementary Fig. 9f ) ( p < 0.01, two-tailed t- test), but down-regulated in 73 Ind OE, 73 Jap Ri, and 71Ri lines (Fig. 3a and Supplementary Fig. 9b, d, e ) ( p < 0.01, two-tailed t- test). The cellular levels of O 2 − and H 2 O 2 were similar to each other in 73 Ind OE, 73 Jap Ri, and 71Ri lines, and were significantly higher compared to WT controls (Fig. 3b–d ), indicating that these lines experienced more severe cold damage than WT plants ( p < 0.01, two-tailed t- test). In contrast, cold damage in leaves of the 71–73 Jap OE lines was significantly milder than in WT plants ( p < 0.01, two-tailed t- test) (Fig. 3b–d ). Fig. 3 Metabolic responses of wild-type and transgenic rice lines under cold stress. a ABA content ( n = 3, 32 plants/replication) and peroxidase (POX) enzyme activity ( n = 8, 10 plants/replication) of transgenic lines under cold stress. b The 3,3’-diaminobenzidine (DAB) and c nitroblue tetrazolium (NBT) staining for the visualization of H 2 O 2 and O 2 − , respectively, in cold-treated rice leaves. Scale bars, 2 mm. d H 2 O 2 content ( n = 8, 10 plants/replication) of transgenic lines under cold stress. OE, overexpression; Ri, RNA interference; 73 Jap , bZIP73 Jap ; 73 Ind , bZIP73 Ind ; 71, bZIP71 ; 71–73 Jap OE, overexpression of both bZIP71 and bZIP73 Jap ; FW, fresh weight. All experiments were conducted using two-week-old seedlings. Error bar, standard deviation; ** p < 0.01, two-tailed t -test Full size image bZIP71 enhances bZIP73 Jap activity to decrease ABA levels ABA plays a critical role in mediating cold stress responses in plants [42] . Under cold stress, increased levels of ABA may help improve cold tolerance of plants. However, since growth and stress responses are two cornerstones of the overall response of plants to the environment [43] , plants under continuous cold stress need to maintain a balance between cold stress adaptation and normal growth, and thus have evolved other mechanisms to avoid over-amplification of the signaling [43] , [44] , [45] . Previous studies indicated that sustained low levels of endogenous ABA could increase seedling tolerance to cold stress [46] , [47] , [48] . To test a potential connection between bZIP73 and ABA, we determined that ABA up-regulated bZIP73 Jap transcription (Supplementary Fig. 4 ), that 73 Jap Ri lines had ABA hypersensitive phenotypes, and that 73 Jap OE lines were neither ABA hypersensitive nor insensitive, while 71–73 Jap OE lines were less sensitive to ABA at the early seedling stage (Supplementary Fig. 10 ). By analyzing promoters of ABA synthesis genes, we identified the two Nine-Cis-Epoxycarotenoid Dioxygenase ( NCED ) ABA synthesis genes OsNCED3 and OsNCED5 as having a G-box motif in their promoters (Supplementary Data 3 ). The in vitro and in vivo interactions between bZIP73 Jap and the promoters of these two genes were verified using ChIP-qPCR and electrophoretic mobility shift assays (EMSA) (Supplementary Fig. 7 ). Furthermore, we found that bZIP71 promotes such interactions in vitro (Supplementary Fig. 7a ). Transient expression assays in rice protoplasts showed that bZIP73 Jap negatively regulates the expression of OsNCED3 and OsNCED5 under cold stress (4 °C, 3 h) (Supplementary Fig. 8 ), and the addition of bZIP71 enhanced the down-regulation (Supplementary Fig. 8 ). Therefore, compared to WT plants, expression levels of OsNCED3 and OsNCED5 and resulting ABA contents in 73 Ind OE, 73 Jap Ri, and 71Ri lines were significantly higher in 2-week-old seedlings after cold treatment (4 °C, 3 h) (Fig. 3a and Supplementary Fig. 9b, d, e ) ( p < 0.01, two-tailed t- test), while those in 71–73 Jap OE lines were significantly lower (Fig. 3a and Supplementary Fig. 9f ) ( p < 0.01, two-tailed t- test). Taken together, these results indicated that bZIP73 Jap mediates cold tolerance by fine-tuning ABA levels, and this activity is enhanced by bZIP71. bZIP73 Ind introgression affects japonica cold tolerance To validate the potential contribution of bZIP73 Jap to cold tolerance in different varieties, we generated a Lemont-background ( japonica ) near-isogenic line (NIL) carrying the bZIP73 Ind allele. The bZIP73 Ind -NIL had a significantly lower survival rate (31.7%) than wild-type Lemont (74.2%) after cold treatment (Fig. 4 ) ( p < 0.01, two-tailed t- test), demonstrating that bZIP73 Jap may be a promising cold tolerance candidate gene for crop breeding. Fig. 4 Increased sensitivity of bZIP73 Ind near-isogenic lines to cold stress. a Cold treatment of bZIP73 Ind near-isogenic lines (NIL) and Lemont ( japonica ) at 8 °C for 6 days and recovery (Recovered) at 28 °C for 7 days. NIL is introgression of bZIP73 Ind into the japonica variety Lemont. b Survival rates of Lemont and NIL after recovery from cold treatment. All data were collected with three biological replicates ( n = 120 each). Error bar, standard deviation. Scale bars, 5 cm; ** p < 0.01, two-tailed t -test in comparisons to the control (Lemont) Full size image bZIP73 has undergone multiple rounds of positive selection Our data suggest that bZIP73 has undergone directional selection in japonica (Supplementary Table 2 ). To further investigate the evolutionary history of bZIP73 , we collected a total of 26 bZIP73 sequences from the Oryza genus. Multiple sequence alignment revealed that the functional polymorphism (FNP, +511) of bZIP73 was differentiated in the rice progenitor O. rufipogon (Fig. 5a , Supplementary Table 3 ). All AA-genome wild rice relatives and 97% of O. rufipogon III (Or-III, the progenitor of temperate japonica [14] ) examined contained the japonica -type bZIP73 allele, indicating that bZIP73 Jap is the ancestral state, while 84% of O. rufipogon I (Or-I, the progenitor of indica [14] ) contained the indica -type allele as the derived state (Fig. 5a , Supplementary Table 3 and Supplementary Data 4 ). As shown by zero heterozygosity and the observed allele frequency of the FNP, the two haplotypes of bZIP73 are nearly fixed in the respective populations of cultivated and common wild rice (Supplementary Table 3 and Supplementary Data 4 ). Fig. 5 Phylogenetic analysis of the bZIP73 gene. a Multiple DNA sequence alignments of 26 OsbZIP73 genes. Nucleotide sequences of the FNP (+511 nt; the first nt of the coding region was defined as +1) are shown. Samples in the green background are cultivated rice; brown background indicates common wild rice O . rufipogon and O. nivara ; gray background indicates other wild rice relatives. Tej, temperate japonica ; trj, tropical japonica , ind, indica ; aro, aromatic ; Or, O. rufipogon . b Phylogenetic network of bZIP73 genes with yellow and pink backgrounds denoting haplotypes carrying the bZIP73 Jap and bZIP73 Ind genotypes, respectively. The size of each node is proportional to the sample size. c – e Haplotype score distributions of AA-genome wild rice ( c ), O. rufipogon ( d ), and cultivated rice ( e ). f Phenotypic distribution of low-temperature seedling survivability (LTSS) of cultivated rice accessions. Arrows indicate the trend of genotypic or phenotypic differentiation Full size image Local reduction of nucleotide diversity ( π ) indicates positive selection. We estimated the nucleotide diversity across a 20 kb genomic region flanking bZIP73 in all rice subpopulations. 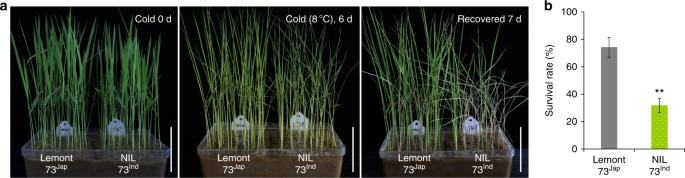Fig. 4 Increased sensitivity ofbZIP73Indnear-isogenic lines to cold stress.aCold treatment ofbZIP73Indnear-isogenic lines (NIL) and Lemont (japonica) at 8 °C for 6 days and recovery (Recovered) at 28 °C for 7 days. NIL is introgression ofbZIP73Indinto thejaponicavariety Lemont.bSurvival rates of Lemont and NIL after recovery from cold treatment. All data were collected with three biological replicates (n= 120 each). Error bar, standard deviation. Scale bars, 5 cm; **p< 0.01, two-tailedt-test in comparisons to the control (Lemont) The nucleotide diversity of bZIP73 was very low in both cultivated ( π < 0.0002) and wild rice ( π < 0.001) populations compared to their genomic backgrounds (~0.002 and ~0.003, respectively [14] ) (Supplementary Table 4 ). Moreover, the diversity of bZIP73 sequences in O. rufipogon III and indica was significantly lower than that of their flanking regions (least significant difference (LSD), α = 0.05, Supplementary Table 4 ), indicating positive selection [49] , [50] . Extended low diversity in flanking regions of japonica bZIP73 indicates a severe bottleneck during the selection of bZIP73 Jap (Supplementary Table 4 ), which might have been completed in O. rufipogon III and was subsequently passed down to japonica . bZIP73 Jap may have facilitated expansion of japonica rice Phylogenetic analysis of bZIP73 suggests that bZIP73 Jap was derived from O. rufipogon III, while bZIP73 Ind was derived from O. rufipogon I (Supplementary Fig. 11 ). The contemporary wild rice may not represent ancestral wild rice before domestication, because it has experienced extensive gene flow from cultivated rice due to open pollination [18] . Moreover, due to the lack of sequence diversity (Supplementary Table 4 ), the phylogeny of bZIP73 fails to reveal binary relationships between rice populations (Supplementary Fig. 11 ). To resolve the reticulated relationships between bZIP73 haplotypes, we constructed a phylogenetic network of bZIP73 . A minimum spanning network (MSN) constructed from 98 haplotypes showed that the two alleles of bZIP73 were derived from distinct common wild rice ecotypes (Fig. 5b ). Similar to what we observed from the nucleotide diversity (Supplementary Table 4 ), the bZIP73 MSN also showed that directional selection of bZIP73 Jap has undergone a more severe bottleneck (fewer steps from prototype to modern haplotype transition), while the bZIP73 Ind haplotype spread gradually with possible gene flow from its direct progenitor O. rufipogon I (Fig. 5b ). Taken together with allele frequency (Supplementary Table 3 ) and phylogeny (Supplementary Fig. 11 ), we conclude parsimoniously that the two alleles of bZIP73 distributed in indica and japonica were derived from different populations of ancestral wild rice. We further mapped the distribution of bZIP73 alleles in our common wild rice samples to environmental factors such as terrestrial temperature. The bZIP73 Ind allele is predominantly distributed in India, Bangladesh, and the west of the Indo-China Peninsula, while the bZIP73 Jap allele is predominant in southern China (Fig. 6 ). Based on our functional studies in cultivated rice, the function of bZIP73 may have also been differentiated in the rice progenitor O. rufipogon . In addition, the average terrestrial temperature in southern China is at least 5 °C lower than that in the geographic distribution areas of bZIP73 Ind (Fig. 6 ), suggesting that the bZIP73 Jap allele may have helped the expansion of cultivated rice progenitors to cooler regions. Strikingly, based on phylogeographic analyses, Huang et al. [14] reported that the common wild rice (Or-III) located in southern China was likely the direct ancestor of japonica [14] , all of which contain the bZIP73 Jap allele as shown in our data (Fig. 6 ). Taken together, the function of the bZIP73 Jap allele may have facilitated the northward expansion of Or-III-like common wild rice to southern China, and may have established a primitive germplasm for the domestication of japonica and its further northward expansion. Fig. 6 Geographic distribution of bZIP73 Jap / Ind in O . rufipogon . The bZIP73 Jap (G) and bZIP73 Ind (A) alleles are labeled in blue and green dots, respectively. Each dot represents the geographic origin of a common wild rice sample. The major geographic distribution of the bZIP73 Ind (A) allele is separated by a black dotted line. Terrestrial surface temperatures averaged from 1960 to 1990 A.D. are shown as a heat map with scale bars in °C. Copyright © Esri. 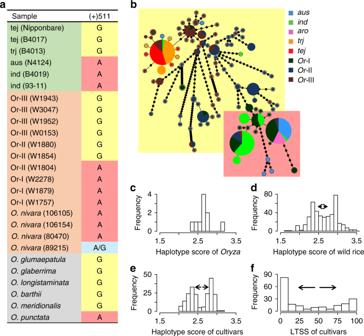Fig. 5 Phylogenetic analysis of thebZIP73gene.aMultiple DNA sequence alignments of 26OsbZIP73genes. Nucleotide sequences of the FNP (+511 nt; the first nt of the coding region was defined as +1) are shown. Samples in the green background are cultivated rice; brown background indicates common wild riceO.rufipogonandO. nivara; gray background indicates other wild rice relatives. Tej,temperate japonica; trj,tropical japonica, ind,indica; aro,aromatic; Or,O. rufipogon.bPhylogenetic network ofbZIP73genes with yellow and pink backgrounds denoting haplotypes carrying thebZIP73JapandbZIP73Indgenotypes, respectively. The size of each node is proportional to the sample size.c–eHaplotype score distributions of AA-genome wild rice (c),O. rufipogon(d), and cultivated rice (e).fPhenotypic distribution of low-temperature seedling survivability (LTSS) of cultivated rice accessions. Arrows indicate the trend of genotypic or phenotypic differentiation All rights reserved Full size image bZIP73 may have undergone balancing selection Our data suggest that the indica genotype of bZIP73 probably underwent positive selection, because bZIP73 Ind is the derived allele (Fig. 5a, b ) that is almost fixed in indica (Supplementary Table 3 and Supplementary Data 4 ), and nucleotide diversity of bZIP73 Ind became locally reduced (Supplementary Table 4 ). Since bZIP73 Jap was selected at the early stage of rice domestication in O. rufipogon III (Supplementary Table 4 ) and further selected in japonica (Supplementary Table 2 ), selection of both bZIP73 genotypes suggests that the gene has undergone balancing selection (Fig. 7 ). Based on the observed lack of heterozygosity (Supplementary Data 4 ) and the mode of spatial distribution of the two alleles (Fig. 6 ), this might have been a location-dependent balancing selection. To further test this hypothesis, we visualized the distribution of haplotype scores estimated from each sample in different populations. A unimodal distribution was observed in AA-genome wild rice (Fig. 5c ), while a bimodal distribution was found for the O. rufipogon population and further enlarged in the cultivated rice population (Fig. 5d, e ), which was also shown by the phenotypic (LTSS) distribution of cultivated rice (Fig. 5f ). Together, these results suggest that artificial selection of bZIP73 was initially started in O. rufipogon III and further fixed in japonica , which may have facilitated the northward expansion of Asian rice, while a second selection event for the indica genotype of bZIP73 occurred later during the balancing selection of bZIP73 (Fig. 7 ). Fig. 7 Step-wise selection model of bZIP73 and the molecular mechanism of bZIP73 Jap -orchestrated cold tolerance in japonica rice Full size image Cold tolerance is an ecologically significant trait for the adaptation of plants to cold climates. In this study, we conducted an association analysis of genomic resequencing data of 91 bZIP genes with LTSS phenotypic data using 203 O . sativa accessions from the USDA rice mini-core collection. By combining it with selective sweep scanning analyses, we found that bZIP73 was the only bZIP gene associated with cold tolerance at the seedling stage that was a target for artificial selection during japonica domestication. Consistently, a bZIP73 Ind NIL in the japonica background was sensitive to cold stress compared to its recurrent japonica parent Lemont (Fig. 4 ). Moreover, bZIP73 Jap RNAi lines enhanced cold sensitivity of japonica rice (Fig. 1 ). These results suggest that bZIP73 Jap is potentially a valuable locus for breeding rice cultivars with superior tolerance to cold stress. Most TFs do not function alone, but rather recruit intermediary proteins (cofactors) for effective initiation of transcription [39] . 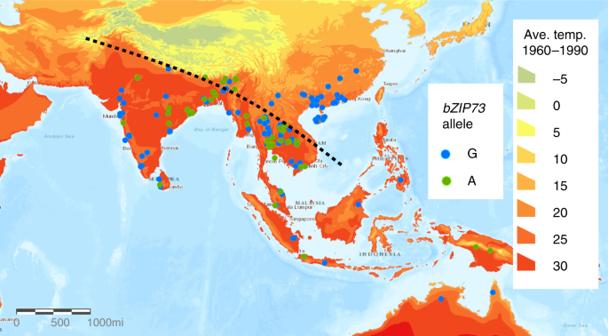Fig. 6 Geographic distribution ofbZIP73Jap/IndinO.rufipogon. ThebZIP73Jap(G) andbZIP73Ind(A) alleles are labeled in blue and green dots, respectively. Each dot represents the geographic origin of a common wild rice sample. The major geographic distribution of thebZIP73Ind(A) allele is separated by a black dotted line. Terrestrial surface temperatures averaged from 1960 to 1990 A.D. are shown as a heat map with scale bars in °C. Copyright © Esri. All rights reserved 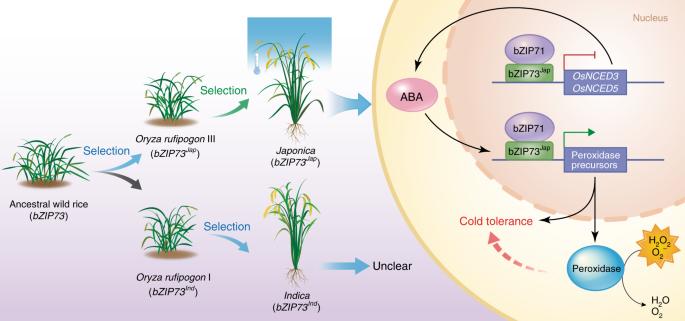Fig. 7 Step-wise selection model ofbZIP73and the molecular mechanism of bZIP73Jap-orchestrated cold tolerance injaponicarice For example, DCA1 acts as a transcriptional co-activator of DST (drought and salt tolerance) and contributes to drought and salt tolerance in rice [39] , while OsbZIP38/LIP19 interacts with OsbZIP87/OBF1 and functions as a cold signal switch in rice [32] . In our study, neither individual 73 Jap OE nor 71OE rice lines had altered cold tolerance, while either bZIP73 Jap or bZIP71 RNAi lines were sensitive to cold stress (Fig. 1 ). We show here that bZIP73 physically interacts with bZIP71 both in vitro and in vivo (Fig. 2 ), and transgenic plants co-expressing bZIP73 Jap and bZIP71 (71–73 Jap OE) are significantly more cold tolerant than WT plants (Fig. 1 ). These results indicate that co-activation of bZIP71-bZIP73 Jap contributes to cold tolerance in rice. bZIP73 Jap trans -activates POX gene precursors under both normal and cold conditions, which can be further enhanced by bZIP71 (Supplementary Fig. 8 ). This enhanced POX activity (Fig. 3a ), together with decreased ROS levels by scavenging H 2 O 2 and O 2 − molecules (Fig. 3 b-d), results in improved cold tolerance of transgenic 71–73 Jap OE lines (Fig. 1 ). In contrast, transgenic lines overexpressing bZIP73 Ind in a japonica background are sensitive to cold stress (Fig. 1 ). This can be explained with a co-dominant-negative scenario in which both bZIP73 Ind and endogenous bZIP73 Jap competitively bind to bZIP71 (Supplementary Fig. 12 ), thus reducing the amount of endogenous bZIP73 Jap -bZIP71 complex and leading to reduced POX activity and increased ROS levels (Fig. 3 ), ultimately causing cold sensitivity of 73 Ind OE lines. In agreement with this, it was previously shown that COLD1 Ind OE lines were less cold tolerant than WT plants as a consequence of competitive binding of COLD1 Ind and COLD1 Jap to RGA1 for regulation of [Ca 2+ ]cyt level and GTPase activity [21] . The bZIP73 Jap gene can be up-regulated by ABA treatment (Supplementary Fig. 4 ); however, bZIP73 Jap represses the two ABA biosynthesis genes OsNCED3 and OsNCED5 during cold treatment (Supplementary Fig. 8 ), leading to lower ABA levels (Fig. 3a ). This indicates that bZIP73 Jap not only responds to ABA signaling, but is also a negative regulator of ABA synthesis and ABA signaling. At the same time, bZIP73 Jap trans -activates POX precursors under both normal and cold temperature conditions (Supplementary Fig. 8 ), thus acting as a positive regulator of ABA-dependent cold stress signaling pathways. Taken together, we propose that bZIP73 Jap is a bi-functional transcription factor with both repressing and activating activities to fine-tune ABA homeostasis and signaling to balance cold stress responses with requirements for growth and development. Similarly, it was shown that OsbZIP23 trans -activates the ABA biosynthesis gene OsNCED4 , leading to higher ABA levels and amplified ABA signaling. Moreover, OsbZIP23 trans -activates the negative regulator of ABA signaling gene PP2C ( OsPP2C49 ) and is also involved in fine-tuning of ABA signaling to promote drought tolerance [44] . Cold tolerance is a very complex trait [3] . Over the past 20 years, extensive efforts were made to identify cold tolerance quantitative trait loci (QTLs) in rice, but only a few associated cold tolerance genes were cloned and functionally verified, such as COLD1 [21] , qCTS12/GSTZ2 [51] , CTB4a [22] , and Ctb1 [52] . Here we show that the japonica allele of bZIP73 associates with the LTSS cold tolerance phenotype of the rice mini-core population, and bZIP71 is associated with the QTL of “survival rate after nature chilling stress” Locus 182 reported by Lv et al. [7] and qLTSS9-1 reported by Schläppi et al. [36] . This suggests that bZIP71 and bZIP73 are two cold tolerance QTL-associated genes that could be used for gene pyramiding to improve cold stress tolerance of rice cultivars. Our evolutionary and population genetic analyses suggest that two specific alleles of bZIP73 were repeatedly selected in both the japonica and indica subspecies of rice, indicating that balancing selection may have occurred for this gene (Fig. 7 ). Association analysis and genome-wide selection screening A total of 91 bZIP genes were collected from Nijhawan et al. [25] and the Michigan State University (MSU) Rice Genome Annotation Project (RGAP) [26] . Whole-genome SNP data including 2.3 million markers were obtained from Wang et al. [34] . SNPs located within the coding sequence (CDS) of bZIP genes with missing data rates less than 80% were retained from the whole-genome dataset. Nucleotide variations of bZIP genes were translated to aa variations using a custom Perl script, which were further screened for minor allele frequency >1% and linkage less than 0.2 using PLINK [53] with parameters –indep-pairwise 5 2 0 . 2 –maf 0 . 01 . Stratification of the USDA mini-core population was performed using the thinned bZIP amino-acid data by PLINK [53] with parameters –cluster –ppc 1e-3 –mds-plot 3 . Gene association analyses with FDR being controlled in multiple testing (FDR_BH) were performed by PLINK [53] using parameters of –covar-number 1,2 –no-fid –no-parents –no-sex –linear –adjust . LTSS phenotype data for mini-core accessions were retrieved from Schläppi et al. [36] . A whole-genome scan for selective sweeps was carried out using OmegaPlus [38] with parameters -minwin 500 -maxwin 25000 -impute N -binary , and the -grid parameter was determined by sequence length with 5 kb per grid. Centromeric regions [26] with 500 kb extended on both sides were masked to control for abnormal LD. Regions with top 5% ω scores in a chromosome were considered being positively selected in the population. bZIP genes that overlapped with or fell into selective sweeps were considered positively selected. Sequences of bZIP73 from wild species and other cultivars bZIP73 orthologs were identified from the genomes of O . barthii , O. glumaepatula , O. glaberrima , O. longistaminata , O. meridionalis , O. punctata , and O. rufipogon using BLAST search in Gramene ( http://www.gramene.org ). Another four orthologs of O . nivara were BLAST-searched from accessions IRGC 106105, IRGC 106154, IRGC 80470, and IRGC 89215 generated by Xu et al. [53] . The other bZIP73 variances were representatives of different accessions of the USDA mini-core collection [34] with IDs indicated in Fig. 5a in parentheses. These varieties were selected based on: (1) the major allele frequency (>80%) of the accession and (2) missing data rate (~6% in average). Multiple sequence alignment of the bZIP73 sequences was performed using MEGA 6.0 with default parameters [54] . DNA constructs and rice transformation Structural information for bZIP73 was obtained from the Plant Transcription Factor Database (PlnTFDB) [55] . For the construction of bZIP73 OE vectors, CDS of bZIP73 genes were reverse transcribed from total RNA extracted from 2-week-old rice seedlings ( bZIP73 Jap from Nipponbare; bZIP73 Ind from Kasalath) using PCR (Supplementary Data 5 ). The sequences were confirmed by PCR fragment sequencing and cloned into binary expression vector pCambia1300-221 to produce 3× Flag-fusion proteins expressed from the strong CaMV 35S promoter, resulting in vectors bZIP73 Jap ::Flag (73 Jap OE) and bZIP73 Ind ::Flag (73 Ind OE). For double overexpression of bZIP71 and bZIP73 Jap (71–73 Jap OE), the coding sequences of bZIP71 and bZIP73 Jap were inserted into the binary expression vector pBWA(V)HS and pBWD(LA)1C, respectively, both of which carried the CaMV 35S promoter and nopaline synthase terminator. The pBWD(LA)1C- bZIP73 Jap construct functioned as the supply vector, and the pBWA(V)HS- bZIP71 construct functioned as the donor vector. Using homologous recombination, the supply vector (pBWD(LA)1C- bZIP73 Jap ) was ligated into the donor vector (pBWA(V)HS- bZIP71 ), generating the pBWA(V)HS- bZIP71 - bZIP73 Jap vector. To generate the bZIP73 -RNAi vector, DNA fragments of bZIP73 (–296 bp to +179 bp) consisting of a sense and antisense strand separated by an intron (the first intron of GA20 oxidase from potato) was inserted into the multiple cloning site of p2300Act (a derivative of pCAMBIA2300 carrying the Actin I promoter and the octopine synthase terminator) [56] . The OE and RNAi constructs were introduced into Agrobacterium tumefaciens strain AGL1 and transformed into the japonica rice cultivar (cv.) Zhonghua 11 (ZH11). All primer sequences are listed in Supplementary Data 5 . Construction of bZIP73 Ind near-isogenic lines A set of chromosome segment substitution lines were constructed by recurrent backcrossing between Teqing ( O. sativa L. ssp. indica ) as the donor parent and Lemont ( O. sativa L. ssp. japonica ) as the recurrent parent. From the BC 1 F 2 to the BC 4 F 2 generation, we continuously selected for target lines containing the recurrent parent markers by using both Simple-Sequence Repeats and Sequence-Tagged Sites markers, and finally a NIL containing bZIP73 Ind was identified in the BC 4 F 2 generation using markers T176 and T183 (Supplementary Data 5 ). The NIL carried an ~615 kb Teqing genome segment containing bZIP73 Ind , and the BC 4 F 6 generation was used in this study. Plant growth conditions and stress treatments All rice transgenic lines used in this study were derived from the japonica cv. ZH11. Seeds were surface sterilized with 70% ethanol for 3 min and soaked in water at 28 °C for 2 days in the dark, then grown hydroponically in the International Rice Research Institute (IRRI) ( http://irri.org/ ) solution in a plant growth chamber (28 °C, 80% relative humidity, and a 14 h day/10 h night photoperiod). Two-week-old seedlings were treated with ABA (100 μM), H 2 O 2 (2 mM), and cold stress (4 °C), respectively. Seedlings were sampled after 0, 0.5, 1, 3, 6, 12, and 24 h of treatment after which total RNA was extracted, and expressions of relative genes were determined using quantitative reverse transcription PCR (qRT-PCR). For cold stress treatment at the seedling stage, homozygous transgenic lines of bZIP73 Jap OE, bZIP73 Ind OE, bZIP71 OE, bZIP71 - bZIP73 Jap OE (71–73 Jap OE), bZIP73 Jap RNAi, bZIP71 RNAi, wild-type ZH11, NIL ( bZIP73 Ind ), and Lemont were used. Two-week-old seedlings were treated at 4 °C for 3 days or 8 °C for 6 days after which plants were allowed to recover at 28 °C for 7 days. All experiments were replicated at least three times. Statistical analyses were performed using the SAS program ( http://www.sas.com ). RNA extraction and quantification Total RNA was prepared from rice tissues using the Trizol reagent (Invitrogen, USA) according to the manufacturer’s protocol. For RT-PCR, 1 μg of total RNA was used for omplementary DNA (cDNA) synthesis using the ReverTra Ace qPCR RT Master Mix and gDNA removal kit (Toyobo, Japan). The obtained cDNA library was used as template for real-time PCR analysis, which was carried out using the SYBR Premix Ex Taq Kit (Takara, Japan) protocol and the ABI PRISM 7900HT Sequence Detection System (Applied Biosystems, USA). The rice Ubiquitin gene ( LOC_Os03g13170 ) was used as internal control. Primer sequences for qRT-PCR are listed in Supplementary Data 5 . The experiments were repeated at least three times. Subcellular localization and trans -activation activity Full-length CDS of bZIP73 Jap and bZIP73 Ind were inserted into pCambia2300-35S-GFP, creating bZIP73 Jap ::GFP and bZIP73 Ind ::GFP fusion vectors. Plasmid DNA was prepared using the Plasmid Midi Kits (Qiagen, Germany) according to the manufacturer’s instructions. Co-transformed bZIP73 Jap/Ind ::GFP and OsMADS3::mCherry vectors were expressed transiently in rice leaf protoplasts using the polyethylene glycol method [57] , [58] . After 12 h of incubation in the dark at 28 °C, green fluorescent protein (GFP) fluorescence was recorded using a confocal laser-scanning microscope (Carl Zeiss, LSM510, Germany). OsMADS3 was used as a nuclear localization marker [59] . Trans -activation activity assays were performed using the Matchmaker GAL4 Two-Hybrid System 3 (Clontech, USA). Full-length coding sequences of bZIP73 Jap , bZIP73 Ind , and a series of truncated sequences of bZIP73 Jap and bZIP73 Ind were amplified, cloned, and fused to the GAL4 DNA-binding domain (BD) in vector pGBKT7 to generate GAL4 BD, BD-73 Jap/Ind (aa: 1–173), BD-73N1 (aa: 1–99), BD-73 Jap/Ind C1 (aa: 100–173), BD-73N2 (aa: 1–156), BD-73M (aa: 77–156), and BD-73 Jap/Ind C2 (aa: 77–173). All constructs and the empty vector were transformed into yeast strain AH109, serially diluted, and spread onto either tryptophan-deficient synthetic dropout medium, or tryptophan-, histidine-, and adenine-deficient synthetic dropout medium. Primer sequences for the constructs are listed in Supplementary Data 5 . Measurement of trans -activation activity in vivo Promoters of OsNCED3 , OsNCED5 , LOC _ Os01g22249 , LOC _ Os03g02920 , LOC _ Os03g32050 , and LOC _ Os04g59210 (~2000 bp upstream of these genes) were amplified and cloned into the pGreenII 0800-LUC vector containing the firefly luciferase (fLUC) gene and the Renilla LUC gene (rLUC) as reporters [60] , while bZIP71 and bZIP73 cDNAs were cloned into the pCambia1300-221-Flag vector as effectors. Assays for transient expression in rice protoplasts were then divided into two populations and incubated for 12 h in the dark. After incubation, one of the transformed protoplast populations was cold treated at 4 °C in the dark for 3 h. Finally, protoplasts were collected by centrifugation at 450 × g for 3 min and immediately utilized for luciferase assays. Luciferase activity was quantified using a dual-luciferase reporter assay kit (Promega, E1910, USA). Five independent transformations for each sample were performed, and the relative luciferase activity was calculated as the ratio of fLUC to rLUC (fLUC/rLUC). Yeast two-hybrid assays cDNA library from various tissues (including roots and shoots at the seedling stage; roots, leaves, stems, flowers, and seeds at the reproductive stage) of rice plants was constructed and detection of interacting proteins was performed using the Make Your Own Mate & Plate™ Library System (Clontech, 630490, USA) and Matchmaker Gold Yeast Two-Hybrid System (Clontech, 630489, USA) following the manufacturer’s instruction. The final prey library was transformed into the yeast strain Y187 following the Yeast Protocols Handbook (Clontech, PT3024-1, USA). The CDS of bZIP73 Jap was cloned into the pGBKT7 vector and functioned as bait. Bait constructs were introduced into yeast strain Y2H Gold (Clontech, 630489, USA). Mating-based yeast two-hybrid assays were performed according to the manufacturer’s instruction (Clontech, 630489, USA) using haploid yeast strains, Y2H Gold and Y187, for bait and prey, respectively. For identification of interaction proteins of bZIP71 and bZIP73 Jap/Ind in yeast, the CDS of bZIP71 was cloned into the pGBKT7 vector and functioned as bait; the CDS of bZIP73 Jap and bZIP73 Ind were, respectively, cloned into the pGADT7 vector and functioned as prey. Bait and prey vectors were co-transformed into the yeast strain Y2H Gold, then incubated on SD/Leu-Trp- plates at 30 °C for 2 days. Positive clones were cultivated on fresh SD/His-Ade-Leu-Trp- plates at 30 °C for 2 to 4 days. β-Galactosidase activity was measured using a liquid culture assay with o -Nitrophenyl-β- d -Galactopyranoside (ONPG, Amresco, USA) as substrate according to the Yeast Protocols Handbook (Clontech, PT3024-1, USA). Primer sequences for vectors are listed in Supplementary Data 5 . Bimolecular fluorescence complementation To perform BiFC assays, CDS of bZIP73 Jap and bZIP73 Ind were cloned into the pSPYNE vector to construct bZIP73 Jap ::NYFP and bZIP73 Ind ::NYFP, and the bZIP71 CDS was cloned into the pSPYCE vector to generate bZIP71::CYFP [61] . Plasmids were transformed into rice protoplasts by polyethylene glycol-mediated transformation [58] , [61] . GFP fluorescence was visualized with a confocal scanning microscope (Carl Zeiss, LSM510, Germany) after incubation in the dark for 14 h. Primer sequences for vectors are listed in Supplementary Data 5 . Co-immunoprecipitation To generate epitope-tagged expression vectors for Co-IP, bZIP73 Jap ::Flag and bZIP73 Ind ::Flag constructs were modified by replacing the 3× Flag with a 6× Myc tag, resulting in bZIP73 Jap ::Myc and bZIP73 Ind ::Myc vectors, respectively. These constructs were introduced into Agrobacterium tumefaciens (AGL1) and transformed into a single-copy homozygous overexpression line of bZIP71::Flag [62] . The Co-IP constructs were also transformed into single-copy homozygous transgenic lines of pCambia1300::Flag (empty binary vector) as the negative control. Soluble proteins were extracted from transgenic lines and Co-IP assays were performed following the protocol of the FLAG Immunoprecipitation Kit (Sigma, FLAGIPT1, USA). Precipitations were visualized on sodium dodecyl sulfate–polyacrylamide gel electrophoresis (SDS-PAGE) using Anti-Flag (Sigma, F1804, USA), Anti-Myc (Sigma, M4439, USA), and horseradish peroxidase (HRP)-conjugated anti-mouse (Promega, W4021, USA) antibodies. All primary antibodies were diluted 1:1000. Primer sequences for vectors are listed in Supplementary Data 5 . The original blot scans are shown in Supplementary Fig. 13 . Pull-down assays The CDS of bZIP71 was cloned into plasmid pGEX4T-3 as a glutathione S -transferase (GST)-fusion protein (GST::bZIP71); bZIP73 Ind was subcloned into maltose-binding protein (MBP) tag containing plasmid pMALc2x to generate fusion protein MBP::bZIP73 Ind . The two fusion proteins were expressed in Escherichia coli BL21. bZIP73 Jap/Ind was subcloned into polyhistidine (His) containing plasmid pET32a to generate fusion proteins of His::bZIP73 Jap/Ind , and fusion proteins were expressed and purified in vitro according to the protocol of the TnT Quick Coupled Transcription/Translation Systems (Promega, USA). Pull-down assays were performed using the MagneGST Pull-Down System (Promega, USA) following the manufacturer’s protocol. For pull-down assays, 2 μg of His::bZIP73 Jap or His::bZIP73 Ind prey proteins were incubated with immobilized GST (2 μg) or GST::bZIP71 (2 μg) bait proteins. For competitive pull-down assays, 2 μg His::bZIP73 Jap and 2, 5, 10 μg MBP::bZIP73 Ind prey proteins were incubated with immobilized GST (2 μg) or GST::bZIP71 (2 μg) bait proteins. Precipitates were washed three times and visualized on SDS-PAGE using Anti-His (GE Healthcare, 27-4710-01, UK), Anti-GST (Beijing Protein Innovation, AbM59001-2H5-PU, China), Anti-MBP (New England Biolab, E8032, USA), and HRP-conjugated anti-mouse (Promega, W4021, USA) antibodies. All primary antibodies were diluted 1:1000. As a control, 10% of precipitation inputs were visualized directly on SDS-PAGE. Primer sequences are provided in Supplementary Data 5 . The original blot scans are shown in Supplementary Fig. 13 and 14 . Chromatin immunoprecipitation assays To perform ChIP assays, 2-week-old seedlings of bZIP73 Jap ::Flag OE, bZIP73 Ind ::Flag OE, and bZIP71 ::Flag OE lines were harvested and immediately fixed with 1% formaldehyde for chromatin isolation. DNA was immunoprecipitated using anti-Flag antibodies and purified using the PCR Purification Kit (Qiagen, Germany) [44] . For ChIP-sequencing, the precipitated and purified DNA from bZIP73 Jap ::Flag OE lines were used to generate sequencing libraries, which were sequenced and processed by Boao Biological Co., Ltd (Beijing, China), generating 19 million 50 bp single-end reads. Raw reads were cleaned and trimmed using a custom Perl script and mapped to the rice reference genome (MSU TIGR v7) [26] . The Model-based Analysis of ChIP-Seq (MACS) software [63] was used to identify chromatin interaction peaks with default parameters. Annotation of the peaks was done using a custom Perl script and all transposon genes were removed. GO enrichment analysis was performed and visualized using the RiceNetDB database [64] . For quantifications using real-time PCR (ChIP-qPCR), the amount of precipitated DNA was calculated relative to the total input chromatin and expressed as percentage of the total according to the formula: % input = 2 Δ C t × 100%, where Δ C t = C t (input)— C t (IP), where C t is the mean threshold cycle of the corresponding PCR reaction. The average expression level was obtained from the percent input values of three replicates [65] . Primer sequences for ChIP-qPCR are listed in Supplementary Data 5 . Electrophoretic mobility shift assays CDS of bZIP71 , bZIP73 Jap , and bZIP73 Ind were amplified and cloned into the pGEX4T-3 vector to generate GST fusion proteins. Vectors of bZIP71 ::GST and bZIP73 Jap ::GST were expressed in E. coli , which were purified following the protocol of the MagneGST Protein Purification System (Promega, USA). The bZIP73 Ind ::GST vector was expressed and purified using the TnT Quick Coupled Transcription/Translation Systems according to the manufacturer’s protocol (Promega, USA). For promoter binding experiments, complementary single-stranded oligonucleotides derived from 70 bp of the G-box region of gene promoters were synthesized as DNA probes. To obtain double-stranded G-Box motif-containing fragments, two complementary oligonucleotides were mixed in a water bath at 95 °C for 5 min and cooled to room temperature for annealing. Mutated G-box was amplified from wild type using mutated primers and was used as negative control. GST fusion protein binding experiments were performed in vitro with the Chemiluminescent EMSA Kit (Beyotime, China) using standard protocols. Primer sequences used are listed in Supplementary Data 5 . Abscisic acid and reactive oxygen species quantifications Peroxidases were extracted in 0.05 M potassium phosphate buffer (pH 7.0) and subsequently centrifuged at 4 °C, 12,000 × g for 15 min. The supernatant was used as the enzyme extract. Measurement of POX activity was performed according to the protocol of the Peroxidase Activity Assay Kit (Beyotime, China). To quantify endogenous ABA, 200 mg of freeze-dried 2-week-old seedlings were extracted twice with 7.5 mL of plant hormone extraction buffer (methanol/water/glacial acetic acid, 80:19:1, v/v/v) supplemented with 20 ng mL −1 2 H 6 ABA internal standards [44] , [66] . Quantifications were performed using an ABI 4000 Q-Trap (Applied Biosystems, USA). ROS examination was carried out using 14-day-old leaves sampled from seedlings with or without cold treatments. The samples were infiltrated with nitroblue tetrazolium (NBT) (Amresco, USA; 1 mg mL −1 NBT in 10 mM sodium azide and 10 mM phosphate buffer, pH 7.8) or 3, 3’-diaminobenzidine (DAB) solutions (Sigma-Aldrich, USA; 1 mg mL −1 DAB-HCl, pH 3.8) [67] . Stained leaves were imaged after removal of chlorophylls by boiling in 95% ethanol for 10 min. H 2 O 2 content in seedlings was detected following the instruction of the Hydrogen Peroxide Assay Kit (Beyotime, China). Phylogenetic reconstruction of bZIP73 A 6-kb SNP dataset spanning bZIP73 (MSU TIGR v7 reference coordinate: Chr9:18121580..18127580) was obtained from the combined population. A total of 452 varieties and accessions of cultivated rice and common wild rice were retained in the dataset after screening for per base missing data rate ≤20% and sequence missing data rate ≤20%. Duplicated sequences from different samples were removed to reduce redundancy. The homologous sequence of the 6-kb region obtained from O. meridionalis was used as outgroup (ROOT). A neighbor-joining (NJ) tree was reconstructed by MEGA 6 [54] using the Jukes–Cantor substitution model with gamma distribution adjustment. A total of 10,000 bootstrap pseudo-replications were conducted; however, due to the lack of diversity in the population sequences, bootstrap supports for branches were very low, indicating that the relationship between branches were not resolved. Thus, bootstrap values were not shown on the NJ tree. Visualization of the NJ tree was done using FigTree v1.4.3 ( http://tree.bio.ed.ac.uk/software/figtree/ ). Reconstruction of the bZIP73 haplotype network Sequences of the 6 kb dataset (missing data rate <30%) were used. Cultivars with admixture backgrounds shown by population structure [18] were removed to reduce noise. A total of 252 sequences were retained with ambiguous loci being imputed using NETWORK 5 ( http://www.fluxus-engineering.com ). A total of 98 haplotypes were identified after the sequence imputation. The MSN of all haplotypes was constructed using Arlequin 3.5.1.2 [68] , visualized using HapStar [69] , and annotated using Inkscape ( www.inkscape.org ). Estimation of haplotype scores was based on the 6 kb SNP markers with minor allele frequency ≥0.2. Genotypes of A, T, C, and G were scored as 1, 2, 3, and 4, respectively, and then the haplotype score was represented by the average of all marker scores. Ortholog sequences of bZIP73 from wild rice relatives were used to estimate the ancestral haplotype score distribution of bZIP73 . The 6 kb regions of O. rufipogon accessions and cultivated rice varieties were used to estimate the progenitor haplotype score distribution and the modern haplotype score distribution, respectively. O. rufipogon samples shown in Fig. 6 were screened for unambiguous +511 SNP genotypes. Global Positioning System (GPS) information of each sample was obtained from Huang et al. [14] and Wang et al. [34] . Maps for sample distributions were created using ArcGIS ® software from the Environmental Systems Research Institute, Inc. (Esri). The map layer of terrestrial temperature averages from 1960 to 1990 A.D. was obtained from ArcAtlas™ ( www.arcgis.com ). Nucleotide diversity of bZIP73 A 20-kb sequence set (Chr9:18112580..18133465) centered on bZIP73 was obtained from the whole-genome dataset with a missing data rate of each sample ≤80%. The whole population was divided into subpopulations representing each rice accession based on the whole-genome phylogenetic tree by Wang et al. [34] . Nucleotide diversity (Tajima’s π ) of each accession was estimated using the script of ThetaPi_v2.pl ( https://github.com/oushujun/ThetaPi ) [70] with parameters -m0 . 8 -w100 -s0 . To detect the local reduction of nucleotide diversity, multiple comparisons of π values of the 4 kb region centered on bZIP73 , the upstream region, and the downstream region were carried out in each subpopulation. The Ryan-Einot-Gabriel-Welsch Q (REGWQ) test and Fisher’s LSD test were applied for non-significant and significant analysis of variance results, respectively. The Satterthwaite approximation was applied for unequal pool sizes. The Kenward–Roger method was applied for unequal variances, and a log transformation was applied where unequal variances could be improved. Statistical analyses were performed using SAS. Data availability ChIP-Seq data that support the findings of this study have been deposited to the NCBI Sequence Read Archive (SRA) under BioProject PRJNA450934 . All other relevant data are freely available from the corresponding author upon request.